The evolution of antisocial punishment in optional public goods games Cooperation, where one individual incurs a cost to help another, is a fundamental building block of the natural world and human society. It has been suggested that costly punishment can promote the evolution of cooperation, with the threat of punishment deterring free-riders. Recent experiments, however, have revealed the existence of 'antisocial' punishment, where non-cooperators punish cooperators. While various theoretical models find that punishment can promote the evolution of cooperation, these models a priori exclude the possibility of antisocial punishment. Here we extend the standard theory of optional public goods games to include the full set of punishment strategies. We find that punishment no longer increases cooperation, and that selection favours substantial levels of antisocial punishment for a wide range of parameters. Furthermore, we conduct behavioural experiments, showing results consistent with our model predictions. As opposed to an altruistic act that promotes cooperation, punishment is mostly a self-interested tool for protecting oneself against potential competitors. Explaining the evolution of cooperation is a topic of importance to both biologists and social scientists, and significant progress has been made in this area [1] , [2] , [3] , [4] , [5] , [6] . Various mechanisms, such as reciprocal altruism, spatial selection, kin selection and multi-level selection, have been proposed to explain the evolution of cooperation. In addition to these mechanisms, the role of costly punishment in promoting cooperation has received much attention. Many behavioural experiments have demonstrated that people are willing to incur costs to punish others [7] , [8] , [9] , [10] , [11] , [12] , [13] , [14] . Complementing these empirical findings, several evolutionary models have been developed to explore the potential effect of punishment on promoting cooperation [15] , [16] , [17] , [18] , [19] , [20] . Many researchers have concluded that the propensity to punish can encourage cooperation, although this position has not gone unquestioned [12] , [21] , [22] , [23] , [24] . The positive role of punishment has been challenged by recent experimental work that shows the existence of a more sinister form of punishment: sometimes non-cooperators punish cooperators [14] , [24] , [25] , [26] , [27] , [28] , [29] , [30] , [31] . In western countries, this 'antisocial punishment' is generally rare, except when it comes in the form of retaliation for punishment received in repeated games [14] , [24] , [25] , [26] , [28] . A series of cross-cultural experiments, however, finds substantial levels of antisocial punishment that cannot be explained by explicit retaliation [27] , [30] , [31] (see Supplementary Notes for additional analysis). It is this general phenomenon of punishment targeted at cooperators, rather than explicit retaliation, which is the focus of our paper. Antisocial punishment is puzzling, as it is inconsistent with both rational self-interest and the hypothesis that punishment facilitates cooperation. Social preference models of economic decision-making also predict that it should not occur [32] , [33] , [34] , [35] . Owing to its seemingly illogical nature, antisocial punishment has been excluded a priori from most previous theoretical models for the evolution of cooperation, which only allow cooperators to punish defectors (exceptions include refs 22 , 23 , 36 , 37 ). Yet empirically, sometimes cooperators are punished, raising interesting evolutionary questions. What are the effects of antisocial punishment on the co-evolution of punishment and cooperation? And can the punishment of cooperators be explained in an evolutionary framework? In this paper, we extend the standard theory of optional Public Goods Games [17] , [18] , [19] , [38] to explore antisocial punishment of cooperators. We study a finite population of N individuals. In each round of the game, groups of size n are randomly drawn from the population to play a one-shot optional public goods game followed by punishment. Each player chooses whether to participate in the public goods game as a cooperator (C) or defector (D), or to abstain from the public goods game and operate as a loner (L). Each cooperator pays a cost c to contribute to the public good, which is multiplied by a factor r >1, and split evenly among all participating players in the group. Loners pay no cost and receive no share of the public good, but instead receive a fixed payoff σ . This loner's payoff is less than the (r−1)c payoff earned in a group of all cooperators, but greater than the 0 payoff earned in a group of all defectors. If only one group member chooses to participate, then all group members receive the loner's payoff σ . Following the public goods game, each player has the opportunity to punish any or all of the n− 1 other members of the group. A given player pays a cost γ for each other player he chooses to punish, and incurs a cost β for each punishment that he receives ( γ < β ). Each of the N players has a strategy, which specifies her action in the public goods game (C, D or L). Each player also has a decision rule for the punishment round that specifies whether she punishes those members of her group who cooperated in the public goods game; those who defected; or those who opted out. A strategy X-Y 1 Y 2 Y 3 is defined by a public goods game action X, and a punishment decision taken towards cooperators Y 1 , defectors Y 2 and loners Y 3 . For example, a C-NPN strategist cooperates in the public goods game, does not punish cooperators, punishes defectors, and does not punish loners; and an L-PNN strategist opts out of the public goods game, punishes cooperators, and does not punish defectors or loners. In total, there are 24 strategies. We contrast this full strategy set with the limited strategy set that has been considered before [17] , [18] , [19] . The limited set has only four strategies: cooperators that never punish, defectors that never punish, loners that never punish, and cooperators that punish defectors. We study the transmission of strategies through an evolutionary process, which can be interpreted either as genetic evolution or as social learning. In both cases, strategies that earn higher payoffs are more likely to spread in the population, whereas lower payoff strategies tend to die out. Novel strategies are introduced by mutation in the case of genetic evolution, or innovation and experimentation in the case of social learning. We use a frequency-dependent Moran process [39] with an exponential payoff function [40] . We perform exact numerical calculations in the limit of low mutation [41] , [42] , which characterizes genetic evolution and the long-term evolution of societal norms, as well as agent-based simulations for higher mutation rates that may be more appropriate for short-term learning and exploration dynamics [19] , [43] ( Supplementary Methods ). In summary, we find that, although punishment dramatically increases cooperation when only cooperators can punish defectors, this positive effect of punishment disappears almost entirely when the full set of punishment strategies is allowed. Just as punishment protects cooperators from invasion by defectors, it also protects defectors from invasion by loners, and loners from invasion by cooperators. Thus punishment is not 'altruistic' or particularly linked to cooperation. Instead, natural selection favours substantial amounts of punishment targeted at all three public goods game actions, including cooperation. Furthermore, we find that the parameter sets that lead to high levels of cooperation (and little antisocial punishment) are those with efficient public goods (large r ) and very weak punishment (small β ). Finally, we generate testable predictions using our evolutionary model, and present preliminary experimental evidence that is consistent with those predictions. Effect of allowing the full set of punishment strategies In the absence of punishment, defectors invade cooperators, loners invade defectors and cooperators invade loners [44] , as in a rock-paper-scissors cycle ( Fig. 1a ). The system spends a similar amount of time in each of the three behavioural states, and cooperation is not the dominant outcome (although there is more cooperation than in the game without loners). If cooperators are allowed to punish defectors, however, the cooperator–defector–loner cycle is broken when the system reaches punishing cooperators ( Fig. 1b ). For this limited strategy set, the population spends the vast majority of its time in a cooperative state [17] . 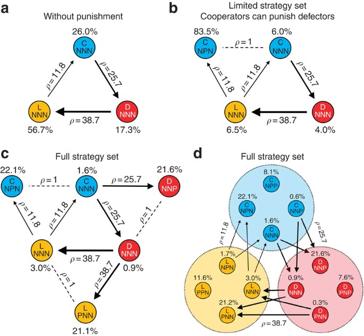Figure 1: Antisocial punishment is common and punishment does not promote cooperation. Time-averaged frequencies of each strategy and transition rates between homogeneous populations, (a) without punishment, (b) when cooperators can punish defectors, and (c,d) with the full set of punishment strategies (for illustrative purposes, only selected strategies are shown in panelc). A strategy X-Y1Y2Y3is defined by a public goods game action (X: C, cooperator; D, defector; L, loner), a punishment decision taken towards cooperators (Y1: N, no action, P, punish), defectors (Y2: N or P) and loners (Y3: N or P). Transition ratesρare the probability that a new mutant goes to fixation multiplied by the population size. We indicate neutral drift (ρ=1, dotted lines), slow transitions (ρ=11.8, thin lines), intermediate transitions (ρ=25.7, medium lines) and fast transitions (ρ=38.7, thick lines). Transitions with rates less than 0.1 are not shown. Parameter values areN=100,n=5,r=3,c=1,γ=0.3,β=1 andσ=1. In panelscandd, strategies that punish others taking the same public goods action are included in the analysis, but not pictured, because they are strongly disfavoured by selection and virtually non-existent in the steady-state distribution. For clarity, transitions with ρ< 10 are not shown in paneld. Figure 1: Antisocial punishment is common and punishment does not promote cooperation. Time-averaged frequencies of each strategy and transition rates between homogeneous populations, ( a ) without punishment, ( b ) when cooperators can punish defectors, and ( c,d ) with the full set of punishment strategies (for illustrative purposes, only selected strategies are shown in panel c ). A strategy X-Y 1 Y 2 Y 3 is defined by a public goods game action (X: C, cooperator; D, defector; L, loner), a punishment decision taken towards cooperators (Y 1 : N, no action, P, punish), defectors (Y 2 : N or P) and loners (Y 3 : N or P). Transition rates ρ are the probability that a new mutant goes to fixation multiplied by the population size. We indicate neutral drift ( ρ= 1, dotted lines), slow transitions ( ρ= 11.8, thin lines), intermediate transitions ( ρ= 25.7, medium lines) and fast transitions ( ρ= 38.7, thick lines). Transitions with rates less than 0.1 are not shown. Parameter values are N= 100, n= 5, r= 3, c= 1, γ= 0.3, β= 1 and σ= 1. In panels c and d , strategies that punish others taking the same public goods action are included in the analysis, but not pictured, because they are strongly disfavoured by selection and virtually non-existent in the steady-state distribution. For clarity, transitions with ρ< 10 are not shown in panel d . Full size image But what happens when all punishment strategies are available? Now the cooperator–defector–loner cycle can be broken as easily in the loner or defector states as in a cooperative state ( Fig. 1c,d ). Without punishment, loners are invaded by cooperators; but loners that punish cooperators are protected from such an invasion. Similarly, defectors are invaded by loners; but defectors who punish loners are protected. Thus, when all punishment strategies are available, the dynamics effectively revert back to the original cooperator–defector–loner cycle. The salient difference is that now the most successful strategies use punishment against threatening invaders. We see that adding punishment does not provide much benefit to cooperators once the option to punish is available to all individuals, instead of being artificially restricted to cooperators punishing defectors. Furthermore, in this light, non-cooperative strategies that pay to punish cooperators seem less surprising, and we see why natural selection can lead to the evolution of antisocial punishment. Robustness to parameter variation These results are not particular to the parameter values used in Figure 1 . We have examined the steady-state frequency of each strategy averaged over 100,000 randomly sampled parameter sets ( Supplementary Notes ). The outcome is remarkably similar to what is observed in Figure 1 . The average level of cooperation is 34% in the absence of punishment, jumps to 87% with restricted punishment, and falls back to 34% with the full punishment strategy set. Although restricted punishment makes cooperation the dominant outcome for the vast majority of parameter sets, the full punishment strategy set does not ( Fig. 2 ). For more than 98% of the randomly chosen parameter sets, the frequency of cooperation is below 0.5 when using the full punishment strategy set. 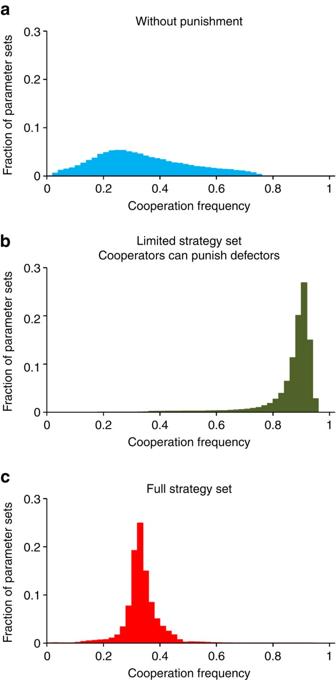Figure 2: Robustness of results across parameter sets. Shown are the results of 100,000 numerical calculations usingN=100,n=5,c=1 and randomly sampling from uniform distributions on the intervals 1 <r< 5, 0 <σ< (r−1)c, 0 <γ< 5, andγ<β< 5γ. Results are shown for (a) the strategy set without punishment, (b) the restricted punishment strategy set where only cooperators can punish loners, and (c) the full punishment strategy set. Figure 2: Robustness of results across parameter sets. Shown are the results of 100,000 numerical calculations using N =100, n =5, c =1 and randomly sampling from uniform distributions on the intervals 1 < r < 5, 0 < σ < ( r −1) c , 0 < γ < 5, and γ < β < 5 γ . Results are shown for ( a ) the strategy set without punishment, ( b ) the restricted punishment strategy set where only cooperators can punish loners, and ( c ) the full punishment strategy set. Full size image We also find that the evolutionary success of antisocial punishment in the full strategy set is robust to variation in the payoff values. The frequencies of all three forms of punishment averaged over the 100,000 parameter sets are quite similar (punish cooperators, 40%; punish defectors, 41%; punish loners, 37%), and the frequency of each punishment type varies relatively little across parameter sets. Furthermore, these results are not unique to the low mutation limit. Agent-based simulations for higher mutation rates show that punishment does not increase the average frequency of cooperation in the full strategy set; and all three forms of punishment (anti-C, anti-D and anti-L) have similar average frequencies ( Supplementary Note ). Here we have shown how evolution can lead to punishment targeted at cooperators. We find that in our framework, loners are largely responsible for this antisocial punishment, and that it protects them against invasion by cooperators. The concept of loners punishing cooperators may seem strange given that loners could be envisioned as trying to avoid interactions with others. However, we find strong selection pressure in favour of such behaviour: loners who avoid others in the context of the public goods game, but subsequently seek out and punish cooperators, outcompete fully solitary loners. We also note that implicit in our framework is some form of information transfer, such as gossip, by which loners are informed of the actions of public goods game participants. Our findings raise questions about the commonly held view that punishment promotes the evolution of cooperation. There is no reason to assume a priori that only cooperators punish others. In fact, there is substantial empirical evidence to the contrary [24] , [25] , [26] , [27] , [28] , [29] , [30] , [31] . As we have shown, using the full strategy set dramatically changes the evolutionary outcome, and punishment no longer increases cooperation. These results highlight the importance of not restricting analysis to a subset of strategies, and emphasize the need to re-examine other models of the co-evolution of punishment and cooperation while including all possible punishment strategies [23] , [36] . But if our framework suggests that the taste for punishment did not evolve to promote cooperation, then why do humans display the desire to punish? And why do many behavioural experiments find that punishment discourages free-riding in the lab [7] , [8] , [9] , [10] , [11] , [12] , [14] ? As opposed to being particularly suited to protecting cooperators from free-riders, our model suggests that costly punishment is an effective tool for subduing potential invaders of any kind. This finding is reminiscent of early work on the ability of punishment to stabilize disadvantageous norms [20] , while adding the critical step of the emergence of punishing behaviour. Our results are also suggestive of a type of in-group bias [45] , [46] , [47] , [48] , [49] , [50] , as our most successful strategists punish those who are different from themselves, while not punishing those who are the same. Therefore, we would expect the level of antisocial punishment to vary depending on the makeup of the population. In populations with a high frequency of cooperators, such as those societies in which most previous behavioural experiments have been conducted, we anticipate punishment to be largely directed towards defectors. In populations where cooperators are less common, however, we expect higher levels of punishment targeted at cooperators. Consistent with this intuition, we find a clear inverse relationship between steady state cooperation frequency and antisocial punishment across randomly sampled parameter sets ( Fig. 3a ). 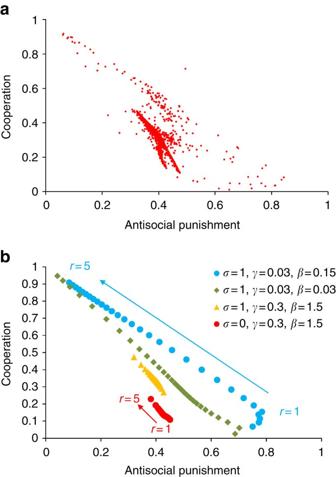Figure 3: Inverse relationship between cooperation and antisocial punishment across parameters. (a) The steady state frequency of cooperation and antisocial punishment from 5,000 random parameter sets is shown. An inverse relationship is clearly visible: when antisocial punishment is rare, cooperation (and pro-social punishment) are common. (b) To explore this relationship, we varyrfrom (σ–c) to 5 for various values ofσ,γ, andβ, fixing N=100,n=5, and c=1. We see that increasingralways increases cooperation while decreasing antisocial punishment. We also see that whenβis small, the range of cooperation and antisocial punishment values is large, whereas values are tightly constrained whenβis larger. Achieving high levels of cooperation and low levels of antisocial punishment requires both large expected returns on public investment (larger) and mostly symbolic punishments (smallβ). Figure 3: Inverse relationship between cooperation and antisocial punishment across parameters. ( a ) The steady state frequency of cooperation and antisocial punishment from 5,000 random parameter sets is shown. An inverse relationship is clearly visible: when antisocial punishment is rare, cooperation (and pro-social punishment) are common. ( b ) To explore this relationship, we vary r from ( σ –c) to 5 for various values of σ , γ , and β , fixing N=100, n =5, and c=1. We see that increasing r always increases cooperation while decreasing antisocial punishment. We also see that when β is small, the range of cooperation and antisocial punishment values is large, whereas values are tightly constrained when β is larger. Achieving high levels of cooperation and low levels of antisocial punishment requires both large expected returns on public investment (large r ) and mostly symbolic punishments (small β ). Full size image Examining specific parameter sets, we find that a larger cooperation multiplier, r , increases cooperation and decreases antisocial punishment ( Fig. 3b ). The importance of r is further demonstrated by a sensitivity analysis calculating the marginal effect of each parameter ( Supplementary Note ). In addition to having large r, we find that punishment must be largely ineffective to achieve a high level of cooperation. Among the parameter sets in Figure 3a with steady state cooperation over 65%, the average effect of punishment is β =0.11 (compared with an overall average of β =7.45). Systematic parameter variation gives further evidence of an interaction between r and β ( Supplementary Note ). When punishment is weak, a wide range of outcomes is possible, including high levels of cooperation if r is large. When punishment is strong, however, all strategies can effectively protect against invasion. Thus neutral drift between punishing and non-punishing strategies dominates the dynamics, and the range of outcomes is tightly constrained. These relationships between cooperation, antisocial punishment and the payoff parameters r and β are consistent with cross-cultural sociological evidence ( Supplementary Note ). Exploring the connection between model parameters, sociological variation and play in experimental games is an important direction for future research across societies. Taken together with data from cross-cultural experiments [27] , [30] , [31] , our evolutionary model generates testable predictions about behaviour in the laboratory. Most previous experiments on public goods have explored compulsory games, which do not offer the choice to abstain in favour of a fixed loner's payoff (an exception is ref. 38 where many people do take the loner's payoff when offered). In the compulsory framework, cross-cultural experiments find evidence of low contributors who punish high contributors. Our model, which is based on an optional public goods game, finds that most punishment of cooperators comes from loners rather than defectors. Therefore, our evolutionary model makes two testable predictions about behaviour in the lab: that many low contributors in compulsory games will opt for the loner's payoff if given the chance, and that players who take the loner's payoff in an optional game will engage in more antisocial punishment in a compulsory game. To begin evaluating these predictions, we use the internet to recruit participants [51] , [52] for two incentivized behavioural experiments [46] , [47] (Methods for experimental details, and Supplementary Note for statistical analysis). In the first experiment, subjects engage in both an optional and a compulsory one-shot public goods game. Consistent with our first theoretical prediction, we find that subjects who choose the loner's payoff in the optional game contribute significantly less in the compulsory game ( Fig. 4a ). Thus many subjects who appear to be defectors in the compulsory game prefer to be loners, and may be bringing intuitions evolved as loners to bear in the experiment. To test our second theoretical prediction, the second experiment recruits subjects to participate in two one-shot public goods games, an optional game followed by a compulsory game with costly punishment. The results are again in agreement with the model's prediction: subjects who opt out of the optional game engage in significantly more punishment of high contributors ( Fig. 4b ). Thus, these experiments provide preliminary empirical evidence in support of our theoretical framework, although intuitions evolved in optional games are not the only possible explanation for the data. Further experimental work exploring cooperation and punishment in optional games, as well as the relationship between play in optional and compulsory games, is an important direction for future research. 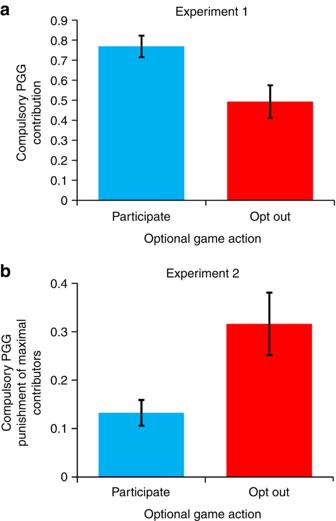Figure 4: Two behavioural experiments are consistent with model predictions. (a) In Experiment 1, subjects play an optional public goods game followed by a compulsory public goods game. The average fraction contributed in the compulsory game is significantly lower among subjects who opt out of the optional game (Rank-sum,N=73,P=0.006). Thus, as predicted, loners contribute less in compulsory games. (b) In Experiment 2, subjects play an optional game followed by a compulsory game with costly punishment. Subjects indicate how much (0, 1 or 2) they would punish each possible contribution level in the compulsory game. Subjects who opt out of the optional game invest significantly more in punishing those that contribute the maximal amount (Rank-sum,N=196,P=0.003). Thus as predicted, loners engage in more antisocial punishment. All games are one-shot interactions among four players, with contributions to the public good multiplied by 2. Punishment technology is 3:1. Results are robust to various controls and alternate methods of analysis;Supplementary Note. Figure 4: Two behavioural experiments are consistent with model predictions. ( a ) In Experiment 1, subjects play an optional public goods game followed by a compulsory public goods game. The average fraction contributed in the compulsory game is significantly lower among subjects who opt out of the optional game (Rank-sum, N =73, P =0.006). Thus, as predicted, loners contribute less in compulsory games. ( b ) In Experiment 2, subjects play an optional game followed by a compulsory game with costly punishment. Subjects indicate how much (0, 1 or 2) they would punish each possible contribution level in the compulsory game. Subjects who opt out of the optional game invest significantly more in punishing those that contribute the maximal amount (Rank-sum, N =196, P =0.003). Thus as predicted, loners engage in more antisocial punishment. All games are one-shot interactions among four players, with contributions to the public good multiplied by 2. Punishment technology is 3:1. Results are robust to various controls and alternate methods of analysis; Supplementary Note . Full size image We have also performed an evolutionary analysis of the compulsory game, where opting out is not possible ( Supplementary Note ). Here we still find that antisocial punishment is favoured by selection; that cooperation and antisocial punishment are inversely correlated; and that non-negligible amounts of pro- and anti-social punishment co-occur in many parameter sets. In the compulsory game, however, cooperation is never favoured over defection using the full strategy set, and antisocial defectors are always the most common strategy. Thus, modelling the game exactly as it is performed in previous compulsory public goods game experiments cannot explain the behaviours that are often observed in such experiments. The preferences displayed by subjects in these experiments therefore seem likely to have evolved under circumstances that are somewhat different from those encountered in the experiments ( Supplementary Note ). Adding the possibility to abstain leads to a model which can describe the range of experimental behaviours. We have shown that although punishment does not increase cooperation or aggregate payoffs in our model, there is nonetheless an incentive to punish. Once punishment becomes available, it is essential for each strategy type to adopt it so as to protect against dominance by similarly armed others. As opposed to shifting the balance of strategies towards cooperation, punishment works to maintain the status quo. This maintenance, however, comes at a high price. Punishment is destructive for all parties and thus reduces the average payoff, without creating the benefit of increased cooperation. If all parties could agree to abandon punishment, everyone would benefit; but in a world without punishment, a strategy that switched to punishing potential invaders would dominate. Therefore, choosing to punish is not altruistic in our framework, but rather self-interested. Punishing leads to a tragedy of the commons where all individuals are forced to adopt punishment strategies. Abstaining from punishment becomes an act of cooperation, while using punishment is a form of second-order defection. The cooperative imperative is not the promotion of punishment, which is costly yet ineffective in our model, but instead the maintenance of cooperation through non-destructive means [12] , [53] , [54] . Experimental overview Together with previous experiments on compulsory games [27] , our model makes testable predictions about the behaviour of experimental subjects: loners are predicted to be lower contributors in compulsory games, and to be most likely to punish high contributors. To evaluate these predictions, we conducted two incentivized behavioural experiments. Experiment 1 investigates the contribution behaviour of loners in a compulsory game, while Experiment 2 considers the degree of antisocial punishment exhibited by loners in a compulsory game. Recruitment using Amazon Mechanical Turk Both experiments were conducted via the internet, using the online labour market Amazon Mechanical Turk (AMT) to recruit subjects. AMT is an online labour market in which employers contract workers to perform short tasks (typically less than 5 min) in exchange for small payments (typically less than $1). The amount paid can be conditioned on the outcome of the task, allowing for performance-dependent payments and incentive-compatible designs. AMT therefore offers an unprecedented tool for quickly and inexpensively recruiting subjects for economic game experiments. Although potential concerns exist regarding conducting experiments over the internet, numerous recent papers have demonstrated the reliability of data gathered using AMT across a range of domains [51] , [52] , [55] , [56] , [57] , [58] . Most relevant for our experiments are two studies using economic games. The first shows quantitative agreement in contribution behaviour in a repeated public goods game between experiments conducted in the physical lab and those conducted using AMT with approximately tenfold lower stakes [58] . The second replication again found quantitative agreement between the lab and AMT, this time in cooperation in a one-shot prisoner's dilemma [51] . It has also been shown that AMT subjects show a level of test–retest reliability similar to what is seen in the traditional physical laboratory on measures of political beliefs, self-esteem, social dominance orientation, and Big-Five personality traits [56] , as well as demographic variables such as belief in God, age, gender, education level and income [52] , [57] ; that AMT subjects do not differ significantly from college undergraduates in terms of attentiveness or basic numeracy skills, and demonstrate similar effect sizes as undergraduates in tasks examining framing effects, the conjunction fallacy and outcome bias [55] ; and are significantly more representative of the American population than undergraduates [56] . Thus, there is ample reason to believe in the validity of experiments conducted using subjects recruited from AMT. Experiment 1 design In October 2010, 124 subjects were recruited through AMT to participate in Experiment 1, and assigned to either a treatment or control condition. Subjects received a $0.20 show-up fee for participating, and earned on average an extra $0.63 on the basis of decisions made in the experiment. First, subjects read a set of instructions for a one-shot public goods game, in which groups of four interact with a cooperation multiplier of r =2, each choosing how much of a $0.40 endowment to contribute (in increments of 2 cents to avoid fractional cent amounts). Subjects then answered two comprehension questions to ensure they understood the payoff structure, and only those who answered correctly were allowed to participate. The 73 subjects randomly assigned to the treatment group were then informed that the game was optional, and they could choose either to participate or to abstain in favour of a fixed payoff of $0.50. Those who chose to participate then indicated their level of contribution. Next, subjects were informed that they would play a second game with three new partners, which was a compulsory version of the first game. They were further informed that one of the two games (optional or compulsory) would be randomly selected to determine their payoff. This was done to keep the payoff range the same as in the control experiment described below, where subjects played only one game. To prevent between-game learning, subjects were not informed about the outcome of the optional game before making their decision in the compulsory game. To test whether behaviour in the compulsory game was affected by the preceding optional game, the remaining 51 subjects participated in a control condition in which they participated only in a compulsory public goods game. Payoffs were determined exactly as described (no deception was used). Experiment 2 design In November 2010, 196 subjects were recruited through AMT to participate in Experiment 2. Subjects received a $0.40 show-up fee for participating, and earned on average an extra $0.92 on the basis of decisions made in the experiment. As in Experiment 1, subjects began by reading a set of instructions for a one-shot public goods game with groups of four, a cooperation multiplier of r =2, and a $0.40 endowment, and then answered two comprehension questions to participate. Subjects were then informed that the game was optional, and that they could choose to participate or opt out for a fixed $0.50 payment. Subjects who chose to participate were given 5 contribution levels to choose from: 0, 10, 20, 30 or 40. Thus, the first game of Experiment 2 is identical to that of Experiment 1's treatment condition, except for a more limited set of contribution options to facilitate punishment decisions as described below. Subjects were then informed that they would play a second game with three new partners, which differed from the first game in two ways: it was compulsory, and it would be followed by a Stage two in which participants could interact directly with each other group member. In Stage two, subjects had three direct actions to pick from: choosing option A had no effect on either player; choosing option B caused them to lose 4 cents while the other player lost 12 cents; and choosing option C caused them to lose 8 cents while the other player lost 24 cents. Thus, we offered mild (B) and severe (C) punishment options with a 1:3 punishment technology. Subjects were allowed to condition their Stage-two choice on the other player's contribution in the compulsory public goods game. To do so, we employed the strategy method: subjects indicated which action (A, B, C) they would take towards group members choosing each possible contribution level (0, 10, 20, 30, 40). It has been shown that using the strategy method to elicit punishment decisions has a quantitative (although not qualitative) effect on the level of punishment targeted at defectors, but has little effect on punishment targeted at cooperators [59] . As antisocial punishment is our main focus, we therefore feel confident in our use of the strategy method. To prevent between-game learning, subjects were not informed about the outcome of the optional game before making their decision in the compulsory game. Payoffs were determined exactly as described (no deception was used). See Supplementary Notes for further details of the experimental setup, the sample instructions and analysis of the experimental results. How to cite this article: Rand, D. G. & Nowak, M. A. The evolution of antisocial punishment in optional public goods games. Nat. Commun. 2:434 doi: 10.1038/ncomms1442 (2011).